Electronic phase separation at the LaAlO3/SrTiO3interface There are many electronic and magnetic properties exhibited by complex oxides. Electronic phase separation (EPS) is one of those, the presence of which can be linked to exotic behaviours, such as colossal magnetoresistance, metal–insulator transition and high-temperature superconductivity. A variety of new and unusual electronic phases at the interfaces between complex oxides, in particular between two non-magnetic insulators LaAlO 3 and SrTiO 3 , have stimulated the oxide community. However, no EPS has been observed in this system despite a theoretical prediction. Here, we report an EPS state at the LaAlO 3 /SrTiO 3 interface, where the interface charges are separated into regions of a quasi-two-dimensional electron gas, a ferromagnetic phase, which persists above room temperature, and a (superconductor like) diamagnetic/paramagnetic phase below 60 K. The EPS is due to the selective occupancy (in the form of 2D-nanoscopic metallic droplets) of interface sub-bands of the nearly degenerate Ti orbital in the SrTiO 3 . The observation of this EPS demonstrates the electronic and magnetic phenomena that can emerge at the interface between complex oxides mediated by the Ti orbital. The perovskite oxides have emerged as one of the most scientifically and technologically interesting material systems. They display a broad range of physical manifestations, including charge-ordered insulator, double-exchange ferromagnet and high-temperature superconductor. Experimental observation of nanoscopic electronic phase separation (EPS) in oxides (for example, underdoped cuprates and doped manganites) in both bulk and thin films [1] , [2] , [3] , [4] , [5] , [6] , [7] , [8] , [9] is of particular interest owing to the speculation that EPS can result in novel electronic properties such as the colossal-magnetoresistive behaviour. In the case of manganites, orbital selective occupancy, Coulomb interaction, Hund's coupling and Jahn–Teller distortions have a significant role in determining the nature of the electronic and magnetic states. The potential of these oxides is further increased by the recent discovery of a variety of new and unusual electronic phases at their interfaces [10] , [11] , [12] , [13] , [14] , [15] , [16] , [17] , [18] , [19] , [20] . A particularly fascinating system is the interface between the perovskite insulators LaAlO 3 and SrTiO 3 , where the existence of a quasi-two-dimensional (quasi-2D) metallic electron layer [13] with signatures of a weak magnetic [14] or a superconducting state [15] , [16] , a metal-to-insulator transition [17] , [18] , correlated electron behaviour [19] and coupled electron hole bilayers [20] has been reported. The electronic properties observed at this interface have been attributed to the electronic reconstruction [13] , [21] that is needed to overcome the diverging Coulomb field of the polar LaAlO 3 layer [22] . Theoretical studies have suggested that the induced interface charges (0.5 e per unit cell) are typically spread over several layers, which correspond to several partially filled sub-bands [23] that can lead to ferromagnetism [24] , [25] , [26] . Caviglia et al . [16] performed electrostatic doping experiments on these superconducting interface samples and successfully modulated their critical temperature ( T c ) but did not observe the existence of ferromagnetism or any other magnetic phase. Recently, Popović et al . [23] have theoretically predicted that the transferred charges at the LaAlO 3 /SrTiO 3 interface occupy nearly ten interface sub-bands. This suggests that EPS is also possible in this system, with most of the charges preferably transferred to a couple of sub-bands in an inhomogeneous fashion. Here, we show evidence for the existence of EPS in this material system. Analyses of electrical, magnetization and magneto-transport data clearly show the separation of the interface charges into a quasi-2D electron gas, ferromagnetic phases persisting above room temperature and strongly diamagnetic and/or paramagnetic phases below 60 K. The EPS is explained on the basis of selective occupancy of interface sub-bands made of the nearly degenerate t 2g orbitals of Ti 3d-states in the SrTiO 3 . Thus, the LaAlO 3 /SrTiO 3 is an active interface the magnetic properties of which can be tailored by processing conditions, temperature and magnetic fields. Sample growth and electronic transport properties LaAlO 3 /SrTiO 3 interfaces were prepared in a wide range of oxygen partial pressures ( P O2 ) from 1×10 −6 to 5×10 −2 mbar (Methods section). The samples fall under two classes, that grown at low pressure and at high pressure. The sheet resistances ( Fig. 1a ) of the samples grown at P O2 ≤10 −5 mbar (low-pressure samples) are ∼ 10 Ω/□ at 300 K and ∼ 1 mΩ/□ at 5 K, with an almost constant carrier density of ∼ 10 17 cm −2 and an increase in mobility to ∼ 10 4 cm 2 V −1 s −1 at 5 K ( Fig. 1b ), which is consistent with earlier reports [13] , [14] , [15] , [16] , [17] , [18] , [19] , [20] , [27] , [28] . The large carrier density of the samples grown in this pressure range indicates a three-dimensional (3D) conductivity that is most likely dominated by oxygen vacancies [28] , [29] , [30] , [31] . The sheet resistances of the samples grown at P O2 ≥10 −4 mbar (high-pressure samples) are 9–13 kΩ/□ at 300 K and gradually decrease to ∼ 200 Ω/□ at 5 K; carrier density ( Fig. 1c ) is reduced by a factor of four from (0.8–1.0)×10 14 cm −2 at 300 K to (2.0–2.5)×10 13 cm −2 at 5 K, indicating significant charge localization. The mobility ( Fig. 1c ) increases significantly to ∼ 10 3 cm 2 V −1 s −1 at 5 K, which suggests that metallic and other (non-conducting) electronic phases coexist. Furthermore, the overall resistivity exhibits metallic behaviour without any discontinuity, despite the change in carrier densities through localization by a factor of four and the mobility enhancement of more than an order of magnitude. 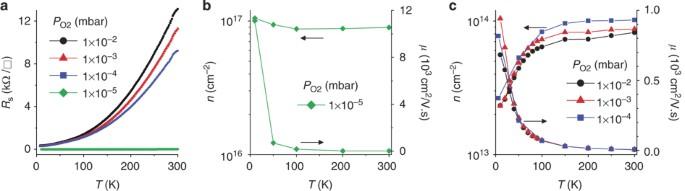Figure 1: Electrical properties. (a) Sheet resistance (Rs) versus temperature (T) of ten unit cells of LaAlO3on SrTiO3prepared at 850 °C under different oxygen partial pressures (PO2) of 10−5, 10−4, 10−3and 10−2mbar, while still maintaining 2D growth. (b) Carrier density (n) and mobility (μ) as a function of temperature for samples prepared at 10−5mbar. (c)nandμas a function of temperature for samples prepared at 10−4, 10−3and 10−2mbar. Figure 1: Electrical properties. ( a ) Sheet resistance ( R s ) versus temperature ( T ) of ten unit cells of LaAlO 3 on SrTiO 3 prepared at 850 °C under different oxygen partial pressures ( P O2 ) of 10 −5 , 10 −4 , 10 −3 and 10 −2 mbar, while still maintaining 2D growth. ( b ) Carrier density ( n ) and mobility ( μ ) as a function of temperature for samples prepared at 10 −5 mbar. ( c ) n and μ as a function of temperature for samples prepared at 10 −4 , 10 −3 and 10 −2 mbar. 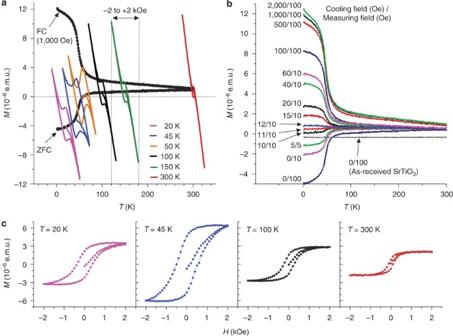Figure 2: Magnetic properties. (a) The 1 kOe FC and ZFC in-plane magnetization (M) data as a function of temperature (T) and measured by a 0.1 kOe magnetic field applied while warming the sample from 2 to 300 K (solid black lines) for the ten unit cells of LaAlO3/SrTiO3samples prepared at an oxygen partial pressure (PO2) of 1×10−2mbar. In a separate measurement after ZFC, ferromagnetic hysteresis loops centred on the diamagnetic branch are observed when sweeping a ±2 kOe magnetic field applied at each temperature. Similar ferromagnetic loops are also observed on the paramagnetic branch when the hysteresis loops are collected after FC (not shown here for clarity). (b) Magnetization as a function of temperature under various cooling temperatures and magnetic fields for the ten unit cells of LaAlO3/SrTiO3samples prepared atPO2=1×10−2mbar. (c) The temperature-dependent ferromagnetic loops inaafter diamagnetic and paramagnetic subtraction. Full size image Magnetic properties Figure 2 summarizes the magnetic properties of the samples grown at P O2 =1×10 −2 mbar. For all the samples described here, the total area of the surface and the volume of the samples are the same (ten unit cells LaAlO 3 on 5×5×0.5 mm 3 SrTiO 3 ). It must be noted that the P O2 under which these films were prepared is at least an order of magnitude higher than those used in previously published reports. Figure 2a shows the zero-field-cooled (ZFC) and field-cooled (FC) magnetization data of the samples as a function of temperature (collected while warming the sample from 2 to 300 K using a small (0.1 kOe) applied magnetic field). For ZFC, a large negative magnetization value indicating a giant diamagnetic response is observed below 60 K, whereas for FC (1 kOe), a positive value, which indicates a paramagnetic response, is seen. In a separate set of measurements, magnetization loops as a function of applied magnetic field (±2 kOe sweep) starting with a positive field were measured at several temperatures. Notably, there is an overlapping ferromagnetic response in addition to the diamagnetic or paramagnetic response, as seen in the form of hysteresis loops extending up to room temperature ( Fig. 2a , also shown in Fig. 2c after background subtraction). In these field sweep curves, the standard temperature-independent diamagnetic contribution of the SrTiO 3 substrate is also discernable. Depending on the cool-down field, the starting point of the hysteresis loops is approximately centered on the diamagnetic (ZFC case) or paramagnetic (FC case) saturation value. Magnetization as a function of temperature under various cooling temperatures and magnetic fields for the ten unit cells of LaAlO 3 /SrTiO 3 samples prepared at P O2 =1×10 −2 mbar is shown in Figure 2b . To rule out any contamination issue, secondary ion mass spectrometric (SIMS) studies were performed, and no evidence of any magnetic element such as Fe, Co, Mn, Ni or Cr was seen in the samples (Methods section). In addition to the electrical data that suggest the coexistence of metallic and other electronic phases, these magnetization data show the coexistence of ferromagnetic phase along with diamagnetic or paramagnetic phases, which support the EPS state at the LaAlO 3 /SrTiO 3 interface. Figure 2: Magnetic properties. ( a ) The 1 kOe FC and ZFC in-plane magnetization ( M ) data as a function of temperature ( T ) and measured by a 0.1 kOe magnetic field applied while warming the sample from 2 to 300 K (solid black lines) for the ten unit cells of LaAlO 3 /SrTiO 3 samples prepared at an oxygen partial pressure ( P O2 ) of 1×10 −2 mbar. In a separate measurement after ZFC, ferromagnetic hysteresis loops centred on the diamagnetic branch are observed when sweeping a ±2 kOe magnetic field applied at each temperature. Similar ferromagnetic loops are also observed on the paramagnetic branch when the hysteresis loops are collected after FC (not shown here for clarity). ( b ) Magnetization as a function of temperature under various cooling temperatures and magnetic fields for the ten unit cells of LaAlO 3 /SrTiO 3 samples prepared at P O2 =1×10 −2 mbar. ( c ) The temperature-dependent ferromagnetic loops in a after diamagnetic and paramagnetic subtraction. Full size image Magnetoresistance Further evidence for the existence of EPS was provided by magnetoresistance (MR) measurements as a function of the angle between the current and field direction. 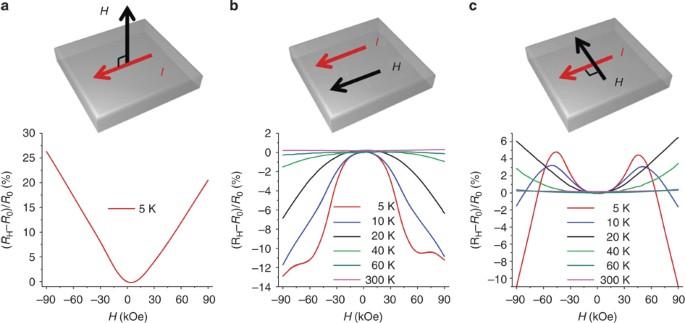Figure 3: MR. The MR, (RH−R0)/R0whereRHis the resistance under a finite magnetic field andR0under zero field, is shown as a function of the applied magnetic fields (H) at different temperatures (T) for three distinct cases as sketched in the insets: (a) magnetic field perpendicular to the current (I) and the substrate surface, (b) magnetic field parallel to the current and the substrate surface and (c) magnetic field parallel to the substrate surface but perpendicular to the current. The results are shown for three different conditions as depicted in Figure 3 : a magnetic field perpendicular to the ab plane of the substrate and current, a magnetic field parallel to the ab plane along the current direction and a magnetic field parallel to the ab plane but perpendicular to the current direction. In the case of magnetic field perpendicular to the ab plane, the cyclotron precession enhances the transit path of the electrons and, if there are electronically phase-separated regions, enhanced scattering of the carriers will occur, resulting in a positive MR (for all temperatures between 5–300 K) that would increase with the magnitude of the field, as is indeed seen in the present case. This supports the idea of phase-separated ferromagnetic regions as opposed to a homogeneous ferromagnetic layer. In the case of a magnetic field parallel to the ab plane along the current direction, there is no cyclotron precession. Instead, alignment of the ferromagnetic regions by the magnetic field makes the scattering more coherent, and hence a negative MR is seen in all applied magnetic fields. This result strongly supports the presence of ferromagnetic scattering centres. In the last case, a magnetic field parallel to the ab plane but perpendicular to the current direction, at low fields, where the electron path is enhanced and incoherent scattering is dominant, a positive MR is seen. At higher fields, the increased coherence of the magnetic regions reduces the electron scattering and a negative MR develops. Hence, the MR data clearly support an EPS scenario involving ferromagnetic regions embedded in a metallic layer. Furthermore, in all cases, the MR values are enhanced significantly at low temperatures with a transition starting at ∼ 60 K, which is in very good agreement with the temperature at which the magnetization value also increases. Figure 3: MR. The MR, ( R H − R 0 )/ R 0 where R H is the resistance under a finite magnetic field and R 0 under zero field, is shown as a function of the applied magnetic fields ( H ) at different temperatures ( T ) for three distinct cases as sketched in the insets: ( a ) magnetic field perpendicular to the current ( I ) and the substrate surface, ( b ) magnetic field parallel to the current and the substrate surface and ( c ) magnetic field parallel to the substrate surface but perpendicular to the current. Full size image Growth pressure dependence The existence of the EPS state critically depends on the LaAlO 3 /SrTiO 3 interface-processing parameters, mainly P O2 . 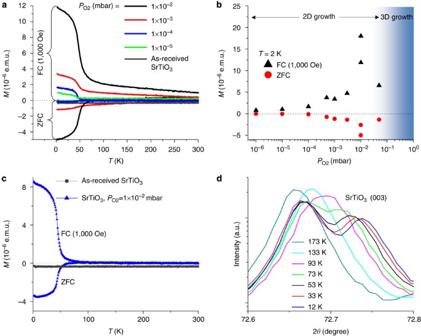Figure 4: Influence of the processing parameters. (a) Magnetization (M) as a function of temperature (T) for samples prepared under different oxygen partial pressures (PO2) of 10−5, 10−4, 10−3and 10−2mbar. (b) The ZFC and FC magnetization data as a function ofPO2conditions. The data were taken while warming the samples from 2 to 300 K in a 0.1 kOe applied magnetic field. (c) The ZFC and FC magnetization data of SrTiO3prepared under conditions similar to those used for the 1×10−2mbar LaAlO3/SrTiO3samples (PO2=1×10−2mbar,T=850 °C). (d) The temperature-dependent X-ray diffraction pattern of SrTiO3show the splitting of the (003) peaks (splitting of other peaks not shown) that appears at temperatures between 73 and 53 K, and grows as the temperature is reduced to 12 K. Figure 4a,b shows the magnetic response of various samples grown at different P O2 . For samples grown at P O2 ≤1×10 −3 mbar, the magnetic responses are much smaller, with an almost unnoticeable transition in the ZFC cases. From the point of view of this paper, the most interesting regime is the high P O2 region, which has not been explored thoroughly until now because it is too close to the 3D growth regime. However, all our samples prepared at P O2 ≤1×10 −2 mbar show clean reflection high-energy electron diffraction (RHEED) oscillations, indicating 2D growth (Methods section). Figure 4: Influence of the processing parameters. ( a ) Magnetization ( M ) as a function of temperature ( T ) for samples prepared under different oxygen partial pressures ( P O2 ) of 10 −5 , 10 −4 , 10 −3 and 10 −2 mbar. ( b ) The ZFC and FC magnetization data as a function of P O2 conditions. The data were taken while warming the samples from 2 to 300 K in a 0.1 kOe applied magnetic field. ( c ) The ZFC and FC magnetization data of SrTiO 3 prepared under conditions similar to those used for the 1×10 −2 mbar LaAlO 3 /SrTiO 3 samples ( P O2 =1×10 −2 mbar, T= 850 °C). ( d ) The temperature-dependent X-ray diffraction pattern of SrTiO 3 show the splitting of the (003) peaks (splitting of other peaks not shown) that appears at temperatures between 73 and 53 K, and grows as the temperature is reduced to 12 K. Full size image Role of SrTiO 3 substrate What is the role of each material in the LaAlO 3 /SrTiO 3 interface structure? To answer this question, we subjected the TiO 2 -terminated SrTiO 3 substrates to identical surface preparation, temperature, oxygen partial pressure and cool-down conditions without deposition of any LaAlO 3 layer on top. Surprisingly, the diamagnetic (ZFC) and paramagnetic (FC) transitions also appeared ( Fig. 4c ) but with values 50% lower than that observed in the LaAlO 3 /SrTiO 3 samples. Furthermore, a tiny magnetic hysteresis loop was seen that was one order of magnitude smaller than that seen in the case of LaAlO 3 /SrTiO 3 . It should be noted that as-received and TiO 2 -terminated SrTiO 3 substrates that are not subjected to the above processing steps show no magnetic effect. Intriguingly, the ∼ 60 K transition temperature below which a very large magnetic response is observed coincides with low-temperature structural phase transitions in SrTiO 3 (tetragonal to orthorhombic at ∼ 65 K and then to rhombohedral at a lower temperature) [32] , [33] . As can be seen in Figure 4d , the temperature-dependent X-ray diffraction data for the samples show that splitting of the SrTiO 3 diffraction peaks starts to appear between 73 and 53 K, and grows as the temperature is reduced to 12 K, indicating phase transformation in SrTiO 3 . This indicates that the surface of the SrTiO 3 and its phase transition are critical for the origin of these magnetic properties and that the role of LaAlO 3 is to significantly amplify these effects via formation of a quasi-2D electron gas at the LaAlO 3 /SrTiO 3 interface. In the following section, we will discuss the possible origin of EPS in this system. Electronic structure calculations by Popović et al . [23] suggest that all the transferred electrons ( ∼ 0.5 e per interface La-atom) are shared by nearly ten interface bands near the Fermi energy. The corresponding charge density is spatially homogeneous in the direction parallel to the interface and quickly decays in the direction perpendicular to the layer. The interface bands are primarily derived from 3 d xy or 3 d xz or 3 d yz orbitals of the Ti atoms. It is known [1] that electron–electron or electron–lattice interactions, Jahn–Teller effects, strain and disorder can modify the band picture considerably and lead to nanoscale charge inhomogeneities. Are we seeing a preferential occupancy of a smaller number of bands, that is, about three out of ten, in a spatially inhomogeneous fashion? Our hypothesis is that transferred charges in a few unit cells of thickness get organized into three states: a quasi-2D dense electron domains (nanoscopic droplets) with a large (superconductor like) diamagnetic moment that have a predominant occupancy in the d xy orbitals, a quasi-2D ferromagnetic nanoscopic regions that have a predominant (close to half filling) occupancy in the ( d yz ) 1 ( d xz ) 1 orbitals and a background of quasi-2D electron gas derived from d xy orbitals. Three possible sources for the high-temperature ferromagnetism are the d xz and d yz orbitals within a single layer provide one-dimensional bands and therefore a larger density of states and corresponding Stoner enhancement, a possibility that 2 e occupy the d xz and d yz orbitals in a spin triplet state and carriers in the d xy permit double exchange similar to that seen in manganites or Ruderman–Kittel–Kasuya–Yosida exchange due to high-mobility electrons. The observed magnetic effects in the treated SrTiO 3 samples can be explained by a migration of electron-like carriers from a finite density of vacancies to the surface of the samples to gain free energies similar to that of the transferred charges at the LaAlO 3 /SrTiO 3 interface. The crucial factor that explains why the three states, that is, ferromagnetic, diamagnetic and/or paramagnetic, and the quasi-2D electron gas can coexist within a few unit cells of the LaAlO 3 /SrTiO 3 interface is their nearly identical free-energy density. The polarization state of SrTiO 3 at nanoscopic scales and other factors, including temperature, control how the interface charges are distributed among the three electron reservoirs. The observation of EPS in this system opens up yet another exciting correlated electron system to scientific study. Besides revealing new phenomena in physics, these unusual magnetic properties may be of use in the fabrication of novel magneto-electronic and tunable magneto-optic devices. Sample growth The LaAlO 3 /SrTiO 3 interfaces were prepared by depositing ten unit cells of LaAlO 3 on a TiO 2 -terminated 0.5-mm-thick SrTiO 3 (001) substrate (double-side polished) in a wide range of P O2 from 1×10 −6 to 5×10 −2 mbar at 850 °C using pulsed laser deposition and a single-crystal LaAlO 3 target. To get single-terminated surfaces, SrTiO 3 was treated with buffered hydrofluoric acid and annealed at 950 °C in oxygen [34] . Using this treatment, an atomically flat SrTiO 3 surface was obtained, as confirmed by atomic force microscopy. The laser pulse (248 nm) energy density was 1.8 J cm −2 and the repetition rate was 1 Hz. During deposition, the film growth was monitored using in situ RHEED, which revealed layer-by-layer growth for samples grown in 1×10 −6 up to 1×10 −2 mbar (close to 3D growth) deposition pressure ( Fig. 5a,b ). For samples grown at 5×10 −2 mbar, the RHEED oscillation started to deviate from normal layer-by-layer growth, indicating an island growth ( Fig. 5c ). After deposition, all samples were cooled to room temperature in oxygen at the deposition pressure. 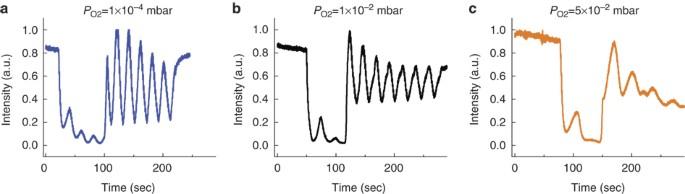Figure 5: Sample growth. RHEED data for samples prepared at oxygen partial pressure (PO2) of (a) 1×10−4mbar and (b) 1×10−2mbar show clean oscillations that indicate 2D growth. (c) A deformed RHEED oscillation for a sample grown at 5×10−2mbar indicates commencement of a 3D growth process. Figure 5: Sample growth. RHEED data for samples prepared at oxygen partial pressure ( P O2 ) of ( a ) 1×10 −4 mbar and ( b ) 1×10 −2 mbar show clean oscillations that indicate 2D growth. ( c ) A deformed RHEED oscillation for a sample grown at 5×10 −2 mbar indicates commencement of a 3D growth process. Full size image Electrical and magnetic measurements The sheet resistance, carrier density and Hall mobility were measured using a Van der Pauw geometry. Before the electrical transport measurements, the magnetic properties of the samples were measured using superconducting quantum interference devices magnetometry. For measurements of the magnetization as a function of temperature, the samples were first cooled to 2 K. The magnetization data were then collected using a series of low magnetic fields ranging from 0.005 to 0.5 kOe during warming from 2 K to room temperature. The magnetic field was applied parallel to the sample surface. SIMS SIMS studies were performed on both magnetic and non-magnetic samples. The SIMS depth profile data ( Fig. 6a ) for the magnetic LaAlO 3 (ten unit cells)/SrTiO 3 sample show that the impurity (including magnetic elements such as Fe, Ni, Co, Cr and Mn) signals are within the measurement noise. The content of magnetic elements in the magnetic LaAlO 3 (ten unit cells)/SrTiO 3 sample and the non-magnetic SrTiO 3 substrate ( Fig. 6b ) was calculated based on relative sensitivity factors from Stevie and Wilson [35] . It is clear that all the impurities in the magnetic and non-magnetic samples is within the noise level, which is at a concentration level of greater than four orders of magnitude lower than the Sr/Ti concentration. Furthermore, the magnetic samples do not show any significant deviation in the concentration of magnetic elements such as Fe, Co, Mn, Ni or Cr compared with the non-magnetic elements. 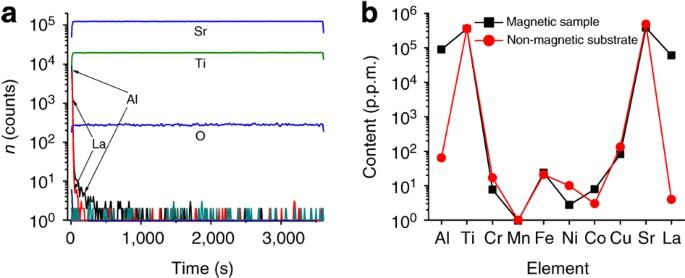Figure 6: SIMS. (a) The SIMS depth profile data for the magnetic LaAlO3(ten unit cells)/SrTiO3show the total counts (n) versus sputtering time for all the detected elements (Sr, Ti, La, Al, B, C, Na, Mg, Si, K, Ca, Cr, Mn, Fe, Ni, Co, Cu, Nb, Ta and Bi). All impurity elements show traces below ten counts. (b) The content of magnetic elements (Cr, Mn, Fe, Ni and Co) in the magnetic LaAlO3(ten unit cells)/SrTiO3sample and the non-magnetic SrTiO3substrate. Figure 6: SIMS. ( a ) The SIMS depth profile data for the magnetic LaAlO 3 (ten unit cells)/SrTiO 3 show the total counts ( n ) versus sputtering time for all the detected elements (Sr, Ti, La, Al, B, C, Na, Mg, Si, K, Ca, Cr, Mn, Fe, Ni, Co, Cu, Nb, Ta and Bi). All impurity elements show traces below ten counts. ( b ) The content of magnetic elements (Cr, Mn, Fe, Ni and Co) in the magnetic LaAlO 3 (ten unit cells)/SrTiO 3 sample and the non-magnetic SrTiO 3 substrate. Full size image How to cite this article: Ariando et al . Electronic phase separation at the LaAlO 3 /SrTiO 3 interface. Nat. Commun. 2:188 doi: 10.1038/ncomms1192 (2011).